Catalysis on singly dispersed bimetallic sites A catalytic site typically consists of one or more atoms of a catalyst surface that arrange into a configuration offering a specific electronic structure for adsorbing or dissociating reactant molecules. The catalytic activity of adjacent bimetallic sites of metallic nanoparticles has been studied previously. An isolated bimetallic site supported on a non-metallic surface could exhibit a distinctly different catalytic performance owing to the cationic state of the singly dispersed bimetallic site and the minimized choices of binding configurations of a reactant molecule compared with continuously packed bimetallic sites. Here we report that isolated Rh 1 Co 3 bimetallic sites exhibit a distinctly different catalytic performance in reduction of nitric oxide with carbon monoxide at low temperature, resulting from strong adsorption of two nitric oxide molecules and a nitrous oxide intermediate on Rh 1 Co 3 sites and following a low-barrier pathway dissociation to dinitrogen and an oxygen atom. This observation suggests a method to develop catalysts with high selectivity. A single reaction event of heterogeneous catalysis occurs on a specific catalytic site at atomic or nanoscale [1] , [2] , [3] . An active catalytic site catalyses a reaction by decreasing its activation barrier through a reaction pathway different from that without a catalyst. Typically, a catalytic site may consist of one, two or a few atoms of surface of a catalyst particle. Atoms of a catalytic site arrange into a configuration that essentially offers a specific electronic structure for the catalytic cycle. Bimetallic nanoparticle catalysts play significant roles in chemical and energy transformations since the second metal (A) could tune catalytic performance of a monometallic catalyst (M) through ligand effect, geometric effect, bi-functional effect or lattice strain effect [2] , [3] , [4] , [5] ( Fig. 1a,b ). Atoms of a catalytic site of a bimetallic nanoparticle could come from more than one element (for example, M and A in Fig. 1c ). Alternatively, they could come from the same element (for example, M in Fig. 1d ) though surface of the bimetallic nanoparticles has both elements M and A. In the latter case, atoms of element A are the modifier of electronic structure but do not directly participate into the catalysis. When metal atoms of a catalytic site come from two different metal elements such as M and A, we term it a ‘bimetallic’ site ( Fig. 1c ); in this case, atoms from both M and A directly participate into the catalytic reaction. One type of such bimetallic sites is referred to M 1 A n (M and A: metal elements, n ≥1), in which both M and A directly participate into a catalytic reaction. The feature of such a bimetallic site is that there is only one atom of M though there is one or more atoms of A. 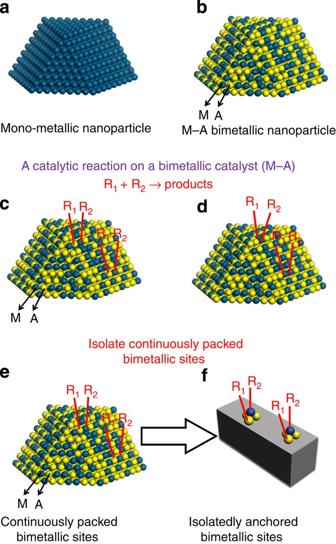Figure 1: Schematic illustration of the isolation of continuous bimetallic sites of alloy nanoparticle to SBMS. Blue and yellow balls represent atoms of metal elements M and A. R1and R2are different reactants. (a) Schematic of a monometallic nanoparticle. (b) Schematic of a bimetallic nanoparticle. (c) Surface of an M–A bimetallic nanoparticle consisting of continuous bimetallic sites; R1and R2bind to A and M atoms, respectively. (d) Surface of an M–A bimetallic nanoparticle consisting of continuous bimetallic sites; however, R1and R2only bind to atoms of metal M instead of A; A is only the modifier of electronic or/and geometric structure. (e) Surface of an M–A bimetallic nanoparticle consisting of continuous bimetallic sites. (f) Isolated bimetallic sites anchored on a non-metallic support; different from the multiple binding configurations of R2on an M–A bimetallic nanoparticle, here R2can only bind to the single atom M through an on-top binding configuration. Figure 1: Schematic illustration of the isolation of continuous bimetallic sites of alloy nanoparticle to SBMS. Blue and yellow balls represent atoms of metal elements M and A. R 1 and R 2 are different reactants. ( a ) Schematic of a monometallic nanoparticle. ( b ) Schematic of a bimetallic nanoparticle. ( c ) Surface of an M–A bimetallic nanoparticle consisting of continuous bimetallic sites; R 1 and R 2 bind to A and M atoms, respectively. ( d ) Surface of an M–A bimetallic nanoparticle consisting of continuous bimetallic sites; however, R 1 and R 2 only bind to atoms of metal M instead of A; A is only the modifier of electronic or/and geometric structure. ( e ) Surface of an M–A bimetallic nanoparticle consisting of continuous bimetallic sites. ( f ) Isolated bimetallic sites anchored on a non-metallic support; different from the multiple binding configurations of R 2 on an M–A bimetallic nanoparticle, here R 2 can only bind to the single atom M through an on-top binding configuration. Full size image Typically, such a bimetallic site, M 1 A n is continuously packed on surface of a bimetallic nanoparticle. Thus, the M 1 A n sites on surface of a bimetallic nanoparticle are at a metallic state. However, if such bimetallic sites (M 1 A n ) are separately anchored on the surface of a non-metallic support such as a transition metal oxide, these isolated bimetallic sites ( Fig. 1f ) are at cationic state. Such isolated bimetallic sites could provide a different surface process including adsorption and dissociation for a reactant molecule or/and an intermediate compared with continuously packed bimetallic sites on a bimetallic nanoparticle. Such a different surface process could facilitate dissociation of a reactant molecule and then accelerate a subsequent coupling with another reactant molecule/dissociated species to form an intermediate or a product molecule. In addition, the single dispersion of atom M of an isolated bimetallic site (M 1 A n ) minimizes choices of potential binding configurations of a reactant molecule, dissociated species, or intermediate on catalyst surface ( Fig. 1f ), in contrast to the potential multiple choices of binding configurations such as on-top, bridge or hollow sites on the surface of a bimetallic nanoparticle. For example, on an M–A bimetallic nanoparticle surface, a R 2 molecule could bind to atop, bridge or even hollow site of M atoms. However, R 2 can bind to M atom through only an atop binding ( Fig. 1f ) on an isolated bimetallic site M 1 A n . Consequently, the minimized choices of binding configurations of reactant, dissociated species or intermediate on isolated M 1 A n sites may enhance catalytic selectivity by following a specific reaction pathway if there are multiple pathways on a bimetallic nanoparticle. Here we report the preparation of a catalyst consisting of singly dispersed bimetallic sites (SBMS) Rh 1 Co 3 through controlled oxidation and reduction processes with the aid of in situ track of evolution of chemistry and structure of the catalyst precursor, and the unique catalytic performance of Rh 1 Co 3 in terms of 100% selectivity for reducing NO to N 2 at 110 °C with a much higher activity than Rh–Co bimetallic nanoparticles at this temperature. Our results illustrate that isolation of bimetallic sites of bimetallic nanoparticles could be used to develop catalysts with higher selectivity or activity. Synthesis of a catalyst of isolated bimetallic sites Rh 1 Co 3 As shown in Fig. 2 , the synthesis of a catalyst of isolated bimetallic sites begins with the formation of hydroxide species M(OH) z on the surface of a reducible oxide A x O y , followed by a calcination at 150 °C in O 2 to anchor M to the surface through formation of M–O–A bonds between singly dispersed M(OH) z species and the surface of the support A x O y , and concluded with a controlled reduction at 300 °C in 5% H 2 to remove some of the oxygen atoms bonded to both atom M 1 and atoms A of the surface, thus forming M–A bonds on the surface of the oxide ( Fig. 2 ). 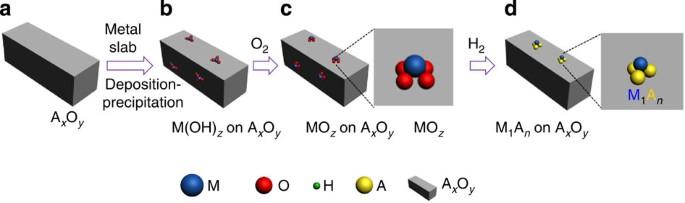Figure 2: Schematic of synthesis of a catalyst of singly dispersed bimetallic sites M1An. (a) Well-crystallized reducible oxide substrate, AxOy. (b) Deposition of hydroxide species of guest metal, M(OH)z, to surface of the oxide support, AxOy; a low concentration of M cations (0. 5 wt% or less) allows them to be singly dispersed on the surface of AxOy; the atomic ratio of M atoms to A atoms of the topmost layer of atoms A of AxOyis typically <5–10%; M(OH)zspecies are weakly bound to the surface of AxOy. (c) Formation of singly dispersed M1Onspecies upon oxidation in 5% O2at 150 °C; M cations are bonded to AxOysurface through M–O–A bonds. (d) A controlled reduction in 5% H2; removal of oxygen atoms between M and A atoms by reduction in H2makes M directly bond with A atoms of oxide support, forming an M1Ansite; as M atoms are singly dispersed on AxOy(due to the low concentration of guest atoms M), the formed M1Anbimetallic sites are isolated. They are called singly dispersed bimetallic sites. Figure 2: Schematic of synthesis of a catalyst of singly dispersed bimetallic sites M 1 A n . ( a ) Well-crystallized reducible oxide substrate, A x O y . ( b ) Deposition of hydroxide species of guest metal, M(OH) z , to surface of the oxide support, A x O y ; a low concentration of M cations (0. 5 wt% or less) allows them to be singly dispersed on the surface of A x O y ; the atomic ratio of M atoms to A atoms of the topmost layer of atoms A of A x O y is typically <5–10%; M(OH) z species are weakly bound to the surface of A x O y . ( c ) Formation of singly dispersed M 1 O n species upon oxidation in 5% O 2 at 150 °C; M cations are bonded to A x O y surface through M–O–A bonds. ( d ) A controlled reduction in 5% H 2 ; removal of oxygen atoms between M and A atoms by reduction in H 2 makes M directly bond with A atoms of oxide support, forming an M 1 A n site; as M atoms are singly dispersed on A x O y (due to the low concentration of guest atoms M), the formed M 1 A n bimetallic sites are isolated. They are called singly dispersed bimetallic sites. Full size image An over-reduction of the support A x O y typically forms an ultrathin bimetallic film of metals M and A; in this case, the guest metal atoms M may alloy with metal atoms of A to form a bimetallic thin layers ( Supplementary Fig. 1 ) instead of isolated M 1 A n bimetallic sites. On the other hand, a less reduction in terms of a reduction at a relatively low temperature could not remove oxygen atoms between M 1 and A of M 1 O n /A x O y ; in this case, the guest metal atom M still bonds to the surface oxygen atoms instead of the surface metal atom(s) A; thus, no bimetallic M 1 A n site is formed. Therefore, an appropriate reduction of the catalyst precursor M 1 O n /A x O y is crucial for the preparation of a catalyst of isolated M 1 A n bimetallic sites, M 1 A n /A x O y . Co 3 O 4 was chosen as one example of oxide support (A x O y ). It generates oxygen vacancies on its surface readily when reduced in a reducing environment [6] , [7] . Reduction of nitric oxide with CO was used as a probing reaction. Co 3 O 4 nanorods were synthesized through a colloidal method [8] , [9] , [10] . Rh atoms were introduced to the surface of Co 3 O 4 nanorods through precipitation of Rh 3+ in the format of Rh(OH) Z species ( Fig. 2b ). Rh(OH) Z weakly binds to the surface of Co 3 O 4 . Evolution of chemical environment of Rh atoms and the surface of cobalt oxide during appropriate oxidation and reduction steps was tracked with an in situ ambient pressure X-ray photoelectron spectroscopy (AP-XPS) [11] . For all in situ studies of this work, data were collected while gaseous reactants remained around a catalyst at a certain temperature. During oxidation in O 2 , Rh atoms are at a cationic state with a high binding energy of Rh 3 d 5/2 at 309.4 eV ( Fig. 3a ) [12] . Upon the formation of Rh 1 O n species on Co 3 O 4 at 150 °C in O 2 , reductions in H 2 at different temperatures were performed. In the reduction at 250 °C in 5% H 2 , Rh 3 d down-shifted by 0.4 to 309.0 eV ( Fig. 3a ). After the reduction in 5% H 2 at 250 °C, a following reduction in H 2 at 300 °C was performed to form isolated bimetallic sites of Rh 1 Co 3 , as is schematically shown in Fig. 2d . During the reduction at 300 °C, Rh 3 d 5/2 further down-shifted by 0.5 eV to 308.5 eV ( Fig. 3a ). Down-shift of binding energy from 309.4 to 308.5 eV clearly suggests a change of the binding environment of Rh atoms during the reduction. The down-shift to 308.5 eV instead of 307.4 eV of metallic Rh shows that Rh atoms of the catalyst upon a reduction at 300 °C in 5% H 2 are not at a metallic state. Figure 4d is the image of HAADF (high-angle annular dark-field) through STEM (scanning transmission electron microscopy) of Rh 1 Co 3 /CoO after catalysis at 400 °C, in which singly dispersed Rh atoms appear as separated spots with high contrast due to the larger atomic number of Rh atoms in contrast to Co (ref. 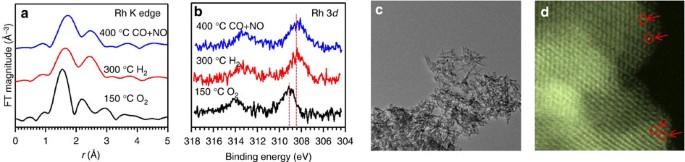Figure 4: Characterizations in the preparation of isolated bimetallic sites. Characterizations in the preparation of isolated bimetallic sites Rh1Co3/CoO and during catalysis byin situEXAFS,in situAP-XPS, andex situHAADF-STEM. (a)r-Space spectra of Rh K edge of catalyst precursor at 150 °C in O2(black line), a following reduction at 300 °C in H2(red line) and during catalysis at 400 °C fromin situEXAFS studies (blue line). (b) Photoemission feature of Rh 3dof catalyst precursor at 150 °C in O2(black line), a following reduction at 300 °C in H2(red line) and during catalysis at 400 °C (blue line) fromin situAP-XPS studies. (c) TEM image (700 × 700 nm) of Rh1Co3/CoO after catalysis. (d) HAADF-STEM image of the catalyst of isolated Rh1Co3bimetallic sites after catalysis at 400 °C; the red arrows mark the Rh atoms that are singly dispersed on CoO. 13 ). This is consistent with the single dispersion of Rh atoms of catalysts after catalysis at 400 °C confirmed with in situ EXAFS ( Fig. 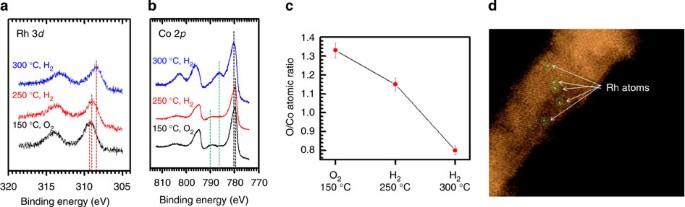4a ). Figure 3:In situstudies of surface chemistry. In situstudies of surface chemistry of the catalyst precursor in the preparation of the catalysts of singly dispersed Rh1Co3bimetallic sites with ambient pressure XPS. (a) Rh 3dphotoemission features during oxidation and reduction processes as marked. (b) Co 2pphotoemission features during oxidation and reduction. (c) Evolution of O/Co atomic ratio under different reaction conditions; the error bar is ±5% of the measured data. (d) HAADF-STEM image (14 × 11 nm) of Rh1Co3/CoO prepared with oxidation at 150 °C in 5% O2and reduction at 300 °C in 5% H2; the bright spots are Rh atoms of Rh1Co3catalytic sites; Rh1Co3sites are singly dispersed. Figure 3: In situ studies of surface chemistry. In situ studies of surface chemistry of the catalyst precursor in the preparation of the catalysts of singly dispersed Rh 1 Co 3 bimetallic sites with ambient pressure XPS. ( a ) Rh 3 d photoemission features during oxidation and reduction processes as marked. ( b ) Co 2 p photoemission features during oxidation and reduction. ( c ) Evolution of O/Co atomic ratio under different reaction conditions; the error bar is ±5% of the measured data. ( d ) HAADF-STEM image (14 × 11 nm) of Rh 1 Co 3 /CoO prepared with oxidation at 150 °C in 5% O 2 and reduction at 300 °C in 5% H 2 ; the bright spots are Rh atoms of Rh 1 Co 3 catalytic sites; Rh 1 Co 3 sites are singly dispersed. Full size image Figure 4: Characterizations in the preparation of isolated bimetallic sites. Characterizations in the preparation of isolated bimetallic sites Rh 1 Co 3 /CoO and during catalysis by in situ EXAFS, in situ AP-XPS, and ex situ HAADF-STEM. ( a ) r -Space spectra of Rh K edge of catalyst precursor at 150 °C in O 2 (black line), a following reduction at 300 °C in H 2 (red line) and during catalysis at 400 °C from in situ EXAFS studies (blue line). ( b ) Photoemission feature of Rh 3 d of catalyst precursor at 150 °C in O 2 (black line), a following reduction at 300 °C in H 2 (red line) and during catalysis at 400 °C (blue line) from in situ AP-XPS studies. ( c ) TEM image (700 × 700 nm) of Rh 1 Co 3 /CoO after catalysis. ( d ) HAADF-STEM image of the catalyst of isolated Rh 1 Co 3 bimetallic sites after catalysis at 400 °C; the red arrows mark the Rh atoms that are singly dispersed on CoO. Full size image In situ EXAFS technique was used to track the evolution of the coordination environment of Rh atoms of the catalyst precursor along the reaction at 150 °C in 5% O 2 , at 300 °C in 5% H 2 and at 400 °C in the mixture of NO and CO ( Fig. 4a , Table 1 and Supplementary Fig. 2 ). The fitted structural parameters of Co and O atoms coordinating to Rh atoms of catalyst particles being annealed at 150 °C in O 2 show that (1) Rh atoms of the catalyst precursor are singly dispersed and (2) these Rh atoms on the cobalt oxide only bond with oxygen atoms with a coordination number of ∼ 4–5 ( Table 1 ). EXAFS study performed on the catalyst upon reduction in 5% H 2 at 300 °C shows that Rh atoms still preserve their single dispersion [CN(Rh–Rh)=0)] and bond with cobalt and oxygen atoms, [CN(Co–Rh)=2.6 and CN(O–Rh)=1.8]. The direct bonding of Rh to Co ( Table 1 ) shows the formation of Rh–Co bonds. Since a Rh atom is isolated from other Rh atoms and bonds with Co atoms, we term the ensemble Rh 1 Co n a singly dispersed bimetallic site or an isolated bimetallic site ( Fig. 2d ). The average coordination number of Co atoms directly bonded to a Rh atom is almost 2 based on EXAFS studies. For simplicity and consistence with the Rh 1 Co 3 structure on CoO proposed through optimization in the following computational studies, Rh 1 Co 3 /CoO is used as the term of this type of isolated bimetallic sites in this communication. Table 1 Coordination numbers and bond lengths. Full size table It is noted that an over-reduction in 5% H 2 at a relatively high temperature of 400 °C forms metallic Co surface layers consisting of a small amount of Rh atoms, as is evidenced by the low binding energy of Co 2 p 3/2 at 778.3 eV and Rh 3 d 5/2 at 307.2 eV ( Supplementary Fig. 1 ). However, AP-XPS studies show that a reduction in 5% H 2 at 250 °C does not form a Rh–Co bond since Rh 3 d 5/2 is still ∼ 309.0 eV instead of 308.5 eV ( Fig. 3 ). Thus, an appropriate reduction temperature is the key for the formation of singly dispersed Rh 1 Co 3 bimetallic sites. Other than the evolution of coordination environment of Rh atoms in the preparation of a catalyst, one obvious change of the support, Co 3 O 4 during reduction at 300 °C in 5% H 2 is the formation of cobalt monoxide in the surface region, evidenced by the observed new peak of Co 2 p 3/2 at 786.4 eV ( Fig. 3b ). This peak is attributed to the characteristic satellite peak of Co 2 p 3/2 of Co 2+ in an octahedral coordination with oxygen atoms in CoO at 786.4 eV (refs 14 , 15 ). Thus, by referring to the characteristic satellite peak of Co 2 p 3/2 of CoO reported in literature [14] , [15] , the photoemission feature of Co 2 p 3/2 collected at 300 °C in 5% H 2 is assigned to CoO. In addition, the formation of CoO is also supported by the O/Co atomic ratio of the catalyst experiencing a reduction at 300 °C in 5% H 2 , 0.80 ( Fig. 3c ), which was measured by taking the stoichiometric ratio of Co 3 O 4 , 1.33 at room temperature as a reference to calibrate the measured atomic ratios (O/Co). As shown in Supplementary Table 1 , the theoretical atomic ratio of all Rh atoms to all Co atoms of the topmost layer of Co atoms of CoO nanoparticles is 1.40%. The measured ratios of the catalyst during catalysis at 150 °C and 400 °C are 1.26 and 1.25%, respectively ( Supplementary Table 1 ), which are quite close to the calculated ideal value, 1.40% ( Supplementary Methods ). These studies suggest that Rh atoms are mainly located on the topmost surface of catalyst particles without obvious thermal diffusion to deep layers. More information on the calculation of these atomic ratios of Rh to Co can be found in Supplementary Methods and Supplementary Figs 11–14 . Catalytic performances of isolated and continuous bimetallic sites After the oxidation of the catalyst precursor in 5% O 2 at 150 °C with a following reduction at 300 °C in 5% H 2 , the catalyst was cooled to 80 °C in 5% H 2 . Once the 5% H 2 was purged, 30 ml min −1 10% CO (balanced with Ar), 20 ml min −1 5% NO (balanced with Ar) and 10 ml min −1 99.999% Ar were mixed and then introduced. Measurements of catalytic performance on the catalyst of isolated Rh 1 Co 3 sites anchored on CoO, Rh 1 Co 3 /CoO were performed in a fixed-bed flow reactor. N 2 O is the by-product of this reaction. Rh 1 Co 3 /CoO exhibits a catalytic selectivity of 100% for the production of N 2 at a temperature as low as 110 °C ( Fig. 5a ). 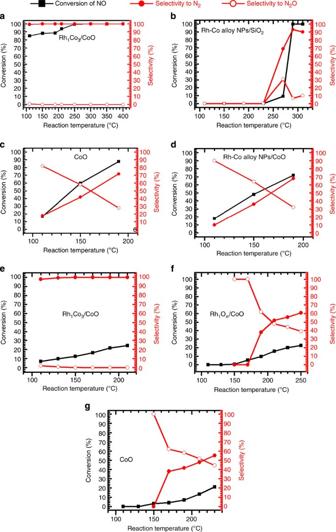Figure 5: Catalytic performances of catalysts measured under different conditions. (a) Rh1Co3/CoO, (b) Rh–Co alloy nanoparticles (2.5 nm) supported on SiO2, (c) pure CoO and (d) Rh–Co bimetallic nanoparticles supported on CoO. Catalytic activity and selectivity of these catalysts (a–d) were measured with the exactly same condition: mixture of 20 ml min−115% NO balanced with Ar, 30 ml min−110% CO and 10 ml min−199.999% Ar; 10 mg of a catalyst was used in each catalytic measurement. (e–g) Catalytic performance 5 mg of Rh1Co3/CoO, 5 mg of Rh1On/CoO and 10 mg of CoO at kinetic controlled region (conversion is lower than 20%); for these measurements in kinetics-controlled regime, 80 ml 15% NO (balanced with Ar) and 12 ml pure CO were mixed and introduced into the reactor. Figure 5: Catalytic performances of catalysts measured under different conditions. ( a ) Rh 1 Co 3 /CoO, ( b ) Rh–Co alloy nanoparticles (2.5 nm) supported on SiO 2 , ( c ) pure CoO and ( d ) Rh–Co bimetallic nanoparticles supported on CoO. Catalytic activity and selectivity of these catalysts ( a – d ) were measured with the exactly same condition: mixture of 20 ml min −1 15% NO balanced with Ar, 30 ml min −1 10% CO and 10 ml min −1 99.999% Ar; 10 mg of a catalyst was used in each catalytic measurement. ( e – g ) Catalytic performance 5 mg of Rh 1 Co 3 /CoO, 5 mg of Rh 1 O n /CoO and 10 mg of CoO at kinetic controlled region (conversion is lower than 20%); for these measurements in kinetics-controlled regime, 80 ml 15% NO (balanced with Ar) and 12 ml pure CO were mixed and introduced into the reactor. Full size image Rh–Co bimetallic nanoparticles supported on SiO 2 , Rh–Co bimetallic nanoparticles supported on CoO and a pure CoO catalyst were prepared with the details described in the section of method. The formation of Rh–Co alloy NP supported on CoO was confirmed with TEM ( Supplementary Fig. 3 ) and XRD ( Supplementary Fig. 4 ). Rh–Co bimetallic nanoparticle supported on SiO 2 is not active at any temperatures <250 °C ( Fig. 5b ). In addition, the activity and selectivity for the production of N 2 on Rh–Co bimetallic nanoparticles supported on CoO at 110 °C are only 20% and 10%, respectively ( Fig. 5d ). Compared with Rh–Co bimetallic nanoparticles supported on CoO, obviously the isolated bimetallic sites Rh 1 Co 3 supported on CoO exhibit an outstanding catalytic performance in terms of high catalytic activity and 100% selectivity for production of N 2 at a temperature as low as 110 °C ( Fig. 5a ). Supplementary Table 2 lists catalytic performances at 110 °C measured under kinetics controlled regime ( Fig. 5e–g ). Clearly, isolated Rh 1 Co 3 bimetallic sites anchored on CoO (Rh 1 Co 3 /CoO) exhibit a much higher activity than Rh–Co bimetallic nanoparticles supported on SiO 2 , pure CoO and Rh–Co bimetallic nanoparticles supported on CoO. It is noted that Rh nanoparticles [16] or Rh-based bimetallic nanoparticles [17] , [18] , [19] , [20] and Rh single crystals [21] are not active at a temperature <240 °C; selectivities for the production of N 2 on Rh nanoparticles at 240 °C (ref. 16 ) and Rh(100) at 255 °C (ref. 21 ) are only ∼ 30% and ∼ 25%, respectively. Overall, the isolated bimetallic sites Rh 1 Co 3 of Rh 1 Co 3 /CoO exhibit an outstanding catalytic performance in terms of quite high catalytic activity and 100% selectivity for the reduction of NO to N 2 at a temperature as low as 110 °C. In situ AP-XPS studies of the catalyst during catalysis at a temperature up to 400 °C showed that Rh atoms of Rh 1 Co 3 /CoO catalyst remains at its oxidizing state ( Fig. 4b ). The high binding energy of Rh 3 d of isolated Rh 1 Co 3 sites anchored on CoO, 308.5 eV, suggests the cationic nature of the Rh atoms in isolated bimetallic sites during catalysis at 400 °C. The preservation of single dispersion of the Rh atoms and the coordination of Co to Rh were supported by in situ studies of EXAFS during catalysis ( Fig. 4a and Table 1 ) and ex situ studies of the catalyst after catalysis at 400 °C using HAADF-STEM ( Fig. 4d ). These characterizations suggest that the isolated bimetallic sites are preserved during catalysis and responsible for the high activity and 100% selectivity for N 2 production. In addition, catalytic performances of Rh 1 Co 3 /CoO and pure CoO under kinetics-controlled regions were measured ( Fig. 5e,g ). By using the number of Rh atoms as the number of Rh 1 Co 3 sites, turnover frequencies (TOFs) of the production of N 2 were calculated and listed in Supplementary Table 2 . The turnover frequency of Rh 1 Co 3 /CoO at 110 °C is 4.4 N 2 molecules per bimetallic site per second. To confirm the importance of direct bonding of Co atoms to a Rh atom in Rh 1 Co 3 /CoO, catalyst Rh 1 O n /CoO was synthesized with the method described in the Methods section. A two-step method was used in the preparation of Rh 1 O n /CoO. CoO substrate was prepared by annealing Co 3 O 4 to 300 °C in 5% H 2 ; the phase transformation was confirmed with XRD; in the second step Rh cations are loaded to the surface of CoO through deposition–precipitation with a following calcination in H 2 at 200 °C for 1 h; the adsorbed Rh(OH) z species were transferred to Rh 1 O n . The existence of Rh atoms on the surface was supported with the preservation of Rh/Co ratio (all Rh atoms to all Co atoms of the topmost layer of Co of CoO) measured with AP-XPS before and after annealing in H 2 at 200 °C. The difference in coordination environment of Rh 1 between Rh 1 Co 3 /CoO and Rh 1 O n /CoO results in a distinct difference in catalytic performance. Figure 5e,f present the catalytic performances of Rh 1 Co 3 /CoO and Rh 1 O n /CoO measured under kinetics-control regime. Rh 1 O n /CoO is not active at a temperature of 150 °C and lower. But Rh 1 Co 3 /CoO is active at 110 °C. In addition, Rh 1 O n /CoO exhibits low selectivity to N 2 production in the temperature range of 150–200 °C. But Rh 1 Co 3 /CoO exhibits a selectivity of 100% for the reduction of NO to N 2 in this temperature range. The distinct difference between Rh 1 O n /CoO and Rh 1 Co 3 /CoO in their catalytic performances results from two factors. One is the difference in geometry; the Rh–O–Co of Rh 1 O n /CoO is different from a bimetallic site of Rh 1 Co 3 /CoO. The existence of a Co–Rh 1 –Co on Rh 1 Co 3 /CoO allows for a strong bonding of two NO molecules (see the following DFT calculations) and thus readily activate NO molecules compared with Rh 1 O n /CoO. Thus, catalyst of singly dispersed bimetallic sites Rh 1 Co 3 is different from the singly dispersed Rh 1 atoms that solely bond to oxygen atoms of the oxide support [22] , [23] , [24] . Location of Rh atoms on CoO To understand the catalytic mechanism of NO reduction with CO on singly dispersed Rh 1 Co 3 anchored on cobalt monoxide, computational modelling of the adsorption, activation and reaction pathway using periodic density functional theory (DFT) was performed. DFT calculations were done for interpretation of the binding environment of Rh atoms ( Fig. 6 ). A Rh atom could anchor to the original position of a missed oxygen (the location of an oxygen vacancy) of CoO in Fig. 6a and thus bond to cobalt atoms; alternatively, it could replace a Co atom of CoO therefore bond to oxygen atoms ( Fig. 6c ). As shown in Fig. 6a , DFT calculations show that the energy change for filling an oxygen vacancy with a Rh atom is −5.39 eV, while the energy change for the replacement of a Co atom with a Rh atom on surface is −3.86 eV. Obviously, filling an oxygen vacancy of CoO with a guest Rh atom is energetically favourable than replacing a Co atom of the surface with a guest Rh atom. This is consistent with the in situ measurements of EXAFS of the catalyst in 5% H 2 at 300 °C showing that Rh atoms bond with Co atoms ( Fig. 4a and Table 1 ). Supplementary Fig. 5b is the optimized structure in which the guest Rh atom fills an oxygen vacancy and thus bonds with three cobalt atoms and one oxygen atom. 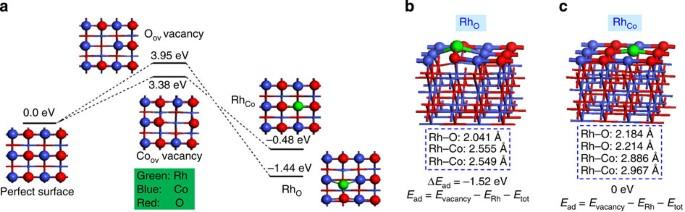Figure 6: Computational studies for understanding the site for anchoring a guest atom, Rh. (a) Evolution of energy of a surface defect (either O vacancy, Ovacor Co vacancy, Covac) while it is filled with a Rh atom. (b) Optimized structure upon filling Rh to oxygen vacancy (RhO); in this case the anchored Rh atom bonds with three cobalt atoms and thus a Rh1Co3bimetallic site is formed. (c) Optimized structure upon replacing a cobalt atom with a Rh atom (RhCo); in this case the anchored Rh atom bonds with four oxygen atoms but not with any cobalt atoms; thus it does not form a Rh1Co3bimetallic site if Rh replaces a Co atom. Figure 6: Computational studies for understanding the site for anchoring a guest atom, Rh. ( a ) Evolution of energy of a surface defect (either O vacancy, O vac or Co vacancy, Co vac ) while it is filled with a Rh atom. ( b ) Optimized structure upon filling Rh to oxygen vacancy (Rh O ); in this case the anchored Rh atom bonds with three cobalt atoms and thus a Rh 1 Co 3 bimetallic site is formed. ( c ) Optimized structure upon replacing a cobalt atom with a Rh atom (Rh Co ); in this case the anchored Rh atom bonds with four oxygen atoms but not with any cobalt atoms; thus it does not form a Rh 1 Co 3 bimetallic site if Rh replaces a Co atom. Full size image Optimization of Rh 1 Co 3 structural model In rock-salt CoO crystal, each Co 2+ is coordinated by six O 2− ions in an octahedral crystal field with Co–O distance of 2.13 Å. The (011) surface of CoO with oxygen vacancies can be viewed as an assembled –O–Co–□–Co–O–Co– chain ( Supplementary Fig. 5a ). When a Rh atom substitutes an oxygen atom on the CoO surface, the Rh 1 atom is not only relocated by 1.13 Å above the vacancy centre (the original oxygen vacancy □, marked with a small light blue ball in Supplementary Fig. 5a ), but also moved closer to an oxygen atom shown as a red ball ( Supplementary Fig. 5b ) in the neighbouring chain with a Rh 1 –O distance of 2.04 Å, which is close to a Co–O single bond estimated as 1.9 Å. As a result, the Rh 1 atom only bonds with one neighbouring O atom, while other O atoms are far from the Rh 1 atom by more than 3.3 Å away. In addition, around a Rh 1 atom, there are three Co atoms Co(3), Co(5), Co(7) marked with stars with a Rh–Co distance averagely 2.54 Å in Supplementary Fig. 5b . However, other three cobalt atoms, Co(2), Co(4) and Co(6) around the Rh 1 atom are far from the Rh 1 at a distance of Rh 1 –Co(2) at 3.15 Å, Rh 1 –Co(4) at 2.81 Å and Rh 1 –Co(6) at 3.15 Å. Therefore, the local coordination shell of Rh 1 atom is referred as Rh 1 Co 3 ; the three Co atoms directly coordinating to Rh 1 of Rh 1 Co 3 are Co(3), Co(5) and Co(7). This optimized geometry model will be used in all the following calculations. Adsorption geometry of NO and CO on Rh 1 Co 3 /CoO As both the surface Rh and Co atoms can adsorb NO and CO, the preferred adsorption models of NO and CO ( Supplementary Fig. 5c–j ) were investigated through DFT calculations. Consistent with the orbital interaction analysis, the NO and CO interact with metal atoms through N- and C-side, respectively. By optimizing the adsorption geometries of NO and CO on various sites with different end-on and bridging binding configurations, the adsorption modes and energies of CO and NO on the surface of a Rh 1 Co 3 /CoO catalyst were evaluated in the DFT calculations. It is found that adsorption of one NO molecule ( Supplementary Fig. 5c ) on Rh 1 atom is slightly more favourable than that of one CO molecule ( Supplementary Fig. 5d ). Because the singly dispersed Rh atom is not saturated in its coordination shell, co-adsorption is in fact more stable than mono-adsorption. Among all the possible co-adsorption models ( Supplementary Fig. 5e–j ), two NO molecules co-adsorbed on the Co–Rh 1 –Co of Rh 1 Co 3 is most stable ( Supplementary Fig. 5e ). Thus, Rh 1 Co 3 adsorbing two NO molecules was used to simulate the reaction pathways and search transition states in the following catalysis studies. Similar to the results for Rh 1 Co 3 /CoO(011), DFT calculations of the adsorption energies of NO, NO+NO, CO+CO or CO+NO on Rh 1 Co 3 /CoO(001) ( Supplementary Fig. 6 ) show that co-adsorption of two NO molecules on Co–Rh 1 –Co of Rh 1 Co 3 /CoO are the strongest adsorption as well. Reaction pathway The reaction pathway was calculated for the reduction of NO with CO on a singly dispersed Rh 1 Co 3 bimetallic site anchored on CoO ( Fig. 7 ). Briefly, the O vac is filled by a single Rh atom to form a singly dispersed bimetallic site Rh 1 Co 3 (step i), which can adsorb two NO molecules on the Co–Rh 1 –Co atoms of a Rh 1 Co 3 site (step ii); two NO molecules couple on Co–Rh 1 –Co to form a N 2 O 2 intermediate (step iii) to facilitate the formation of intermediate N 2 O; meanwhile one CO molecule can adsorb on the Co atom neighbouring to Rh 1 Co 3 (step iv). 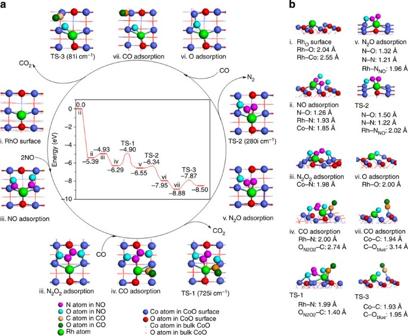Figure 7: Reaction pathway. Reaction pathway for reduction of NO with CO on the singly dispersed Rh1Co3supported on CoO proposed from DFT calculations. (a) Reaction pathway and energy profile. (b) Calculated structural parameters of intermediates and transition states in the pathway. Figure 7: Reaction pathway. Reaction pathway for reduction of NO with CO on the singly dispersed Rh 1 Co 3 supported on CoO proposed from DFT calculations. ( a ) Reaction pathway and energy profile. ( b ) Calculated structural parameters of intermediates and transition states in the pathway. Full size image The first CO 2 molecule is released after the adsorbed CO molecule couples with one O atom of N 2 O 2 adsorbed on the Co–Rh 1 –Co site ( TS-1 ). This coupling yields a CO 2 molecule and forms an intermediate N 2 O remaining on the surface (step v). It is noted that the N–O bond in the intermediate N 2 O stretches to form a transition state with a small barrier of 0.21 eV ( TS-2 ), which leads to a ready cleavage of N–O bond of the intermediate N 2 O and then releases a N 2 molecule and leaves an O atom on Rh 1 (step vi). By adsorbing a second CO on a nearby Co atom (step vii) and then coupling to the left oxygen atoms on the Rh 1 atom, a second CO 2 molecule is released from the surface; thus a catalytic cycle is finished. In this catalytic cycle, the catalyst releases two CO 2 molecules and one N 2 molecule and then recovers its original surface structure (step i in Fig. 7 ). The inset of Fig. 7a presents the calculated energy profile with the partially reduced system as the reference for the energies in eV. Figure 7b lists the calculated structural parameters of intermediates and transition states of this pathway. In this reaction pathway, the Rh 1 Co 3 site plays a crucial role in the high activity and selectivity in reducing NO with CO. The local coordination environment of the bimetallic site Rh 1 Co 3 helps to activate the two NO molecules on Co–Rh 1 –Co of Rh 1 Co 3 through co-adsorption and coupling. The catalytic elementary steps, evolution of energies and activation barriers are listed in Table 2 . Especially noteworthy is the extremely low activation barrier of N 2 O decomposition (0.21 eV) to a N 2 molecule on the Rh 1 Co 3 /CoO catalyst. Given the high reaction temperature, this step is virtually barrierless in terms of Gibbs free energies. Thus, these calculation results are quite consistent with the fact that the catalyst of Rh 1 Co 3 bimetallic sites is active at a temperature as low as 110 °C with a selectivity of 100% for production of N 2 . Table 2 Process energies and activation barriers. Full size table Other than the formation of a N 2 molecule through breaking N–O bond of the intermediate N 2 O (v of Fig. 7 ), we further considered other pathways. For instance, N atom formed through dissociation of one of the two NO molecules (i of Supplementary Fig. 7 ) could couple with a N atom of another NO molecule that bonds to an oxygen vacancy through the oxygen atom of NO (ii of Supplementary Fig. 7 ); this coupling weakens N–O bond of the adsorbed NO molecule and thus forms a N 2 species strongly adsorbed on the Rh atom with a quite high adsorption energy (iv of Supplementary Fig. 7 ). The barrier of the transition state (iii of Supplementary Fig. 7 ) to form N 2 molecule is 0.5 eV. However, the binding energy of N 2 molecule on Rh atom is quite large (iv of Supplementary Fig. 7 ), which makes this pathway less favourable. To understand the difference in binding of NO molecules on isolated sites Rh 1 Co 3 supported on CoO and surface of a Rh–Co bimetallic nanoparticle supported on CoO, structural models of Rh 1 Co 3 /CoO with one adsorbed NO molecule ( Supplementary Fig. 8a ) and Rh–Co bimetallic nanoparticle/CoO with one adsorbed NO molecule ( Supplementary Fig. 8b ) were built. DFT calculations show that adsorption of a NO molecule on Rh atom of Rh 1 Co 3 is definitely stronger than that on a zero-valent Rh(0) atom of a Rh–Co bimetallic nanoparticle ( Supplementary Table 3 ). Consistent with this difference, the calculated N····Rh distance of Rh 1 Co 3 /CoO is ∼ 0.03 Å smaller in contrast to that of Rh–Co bimetallic nanoparticle/CoO. These differences suggest that the Rh 1 Co 3 /CoO catalyst can readily activate NO compared with Rh–Co bimetallic nanoparticle/CoO. The computed electron density difference maps of the two different fragments on Rh 1 Co 3 /CoO and Rh–Co bimetallic nanoparticle/CoO are shown in Supplementary Fig. 8c and d , respectively. In these plots ( Supplementary Fig. 8c and d ), a decrease in electron density is shown in blue, electron enrichment indicated in red; white region indicates little change in electron density. The more red colour between N and Rh in Rh 1 Co 3 /CoO ( Supplementary Fig. 8c ) than the one in the Rh–Co bimetallic nanoparticle supported on CoO ( Supplementary Fig. 8d ) shows that the Rh–N bond on Rh 1 Co 3 /CoO is stronger than that on Rh–Co nanoparticles supported on CoO. Thus the charge transfer from NO to Rh atoms of Rh 1 Co 3 /CoO is larger than that on Rh–Co bimetallic nanoparticle/CoO. The calculated Bader charges ( Supplementary Table 4 ) revealed that the Rh 1 single atom of Rh 1 Co 3 /CoO carries positive charge upon adsorption of NO while the Rh atom in Rh–Co alloy NP/CoO carries negative charge upon NO adsorption. The positive charge on Rh 1 of a singly dispersed Rh 1 Co 3 site allows more electron transfer from NO, which enhances the Rh–N bond and thus largely weakens the N–O bond of NO molecule on Rh 1 Co 3 . The spin-polarized projected density of states (PDOS) of the 4 d states of Rh atom and the N-2 p and O-2 p orbitals of adsorbed NO on Rh 1 Co 3 /CoO and Rh–Co bimetallic nanoparticle/CoO are shown in Supplementary Fig. 8e and f , respectively. The spin-polarized projected density of states show that below the Fermi level ( E F ) Rh 4 d states in Rh 1 Co 3 /CoO catalyst are more localized than the Rh 4 d states in Rh–Co bimetallic nanoparticle/CoO. In addition, Rh 4 d states in Rh 1 Co 3 /CoO ( Supplementary Fig. 8e ) are mixed better with N 2 p and O 2 p states than Rh 4 d states in Rh–Co bimetallic nanoparticle/CoO ( Supplementary Fig. 8f ), indicating a strong interaction between Rh 1 atom of Rh 1 Co 3 and the adsorbed NO molecule. One critical difference between a singly dispersed Rh 1 Co 3 site anchored on CoO and a Rh–Co bimetallic nanoparticle supported on CoO is the 100% selectivity for production of N 2 in reduction of NO with CO on Rh 1 Co 3 ( Fig. 5a ). On Rh–Co bimetallic nanoparticle supported on CoO ( Fig. 5d ), however, selectivity for production of N 2 is only 10%. To understand this difference in catalytic selectivity for production of N 2 O on the two surfaces, structural models of Rh 1 Co 3 /CoO and Rh–Co bimetallic nanoparticle/CoO ( Supplementary Fig. 9 ) were built. The calculated adsorption energies of N 2 O for Rh 1 Co 3 /CoO and Rh–Co bimetallic nanoparticles/CoO are −1.56 and −0.85 eV, respectively. N 2 O is the by-product of the reduction of NO with CO; it is also the intermediate for production of N 2 (step 5 in Table 2 ). A stronger binding of N 2 O prevents it from molecular desorption. Thus, the selectivity for the production of N 2 O on Rh 1 Co 3 /CoO is low since the adsorption of N 2 O on Rh 1 Co 3 /CoO is stronger than that on Rh–Co bimetallic nanoparticle/CoO. In addition, as the activation barrier for dissociating N 2 O to N 2 and O on Rh 1 Co 3 /CoO is only 0.21 eV ( TS- 2 in Fig. 7 ), N 2 O can readily dissociate to N 2 on Rh 1 Co 3 /CoO at a relatively low temperature. Overall, the stronger binding of N 2 O on Rh 1 Co 3 site and the rather low activation barrier for dissociation of the intermediate N 2 O to N 2 on Rh 1 Co 3 /CoO, make the reduction of NO to N 2 with a high selectivity at a relatively low temperature in contrast to Rh–Co bimetallic nanoparticles/CoO. As described in literature [25] , the test temperature of engine of a gasoline vehicle is 1,100 °F (593 °C), stability tests by measurements of conversion and selectivity of the catalyst, Rh 1 Co 3 /CoO were performed. Concerning the real hydrothermal conditions in a three-way catalytic reactor, water vapour was also introduced to the reactor to simulate the exhaust of gasoline engines. As shown in literature [26] , typically the composition of water vapour is 20 times of nitric oxide and carbon monoxide. Thus, stability of 10 mg catalyst was tested in a mixture of 12 ml min −1 NO, 12 ml min −1 CO, 68 ml min −1 Ar and H 2 O vapour generated from 0.18 ml min −1 water were mixed and then introduced to a fixed-bed flow reactor. The molar ratio of NO:CO:H 2 O is 1:1:20. The conversion and selectivity of this catalyst remained nearly constant within 168 h. These studies suggest that the isolation of bimetallic sites on non-metallic supports is a promising approach for developing catalysts, since such centres exhibit cationic states and offer the fewest binding configurations for reactant molecules—distinctly different from bimetallic nanoparticles. Preparation of isolated Rh 1 Co 3 sites on cobalt oxide Co 3 O 4 nanorods were synthesized with a modified wet chemistry method in literature [27] . To synthesize a catalyst of singly dispersed Rh 1 Co 3 sites, Co 3 O 4 nanorods were synthesized with a modified wet chemistry method and a following calcination at high temperature [27] , [28] . Then, species of rhodium precursor were introduced on the crystallized Co 3 O 4 nanorods through a deposition–precipitation with a mass ratio of Rh to Co 3 O 4 of 0.25 wt%. Rh(NO 3 ) 3 (Sigma-Aldrich, ∼ 36% Rh basis; 0.28 g) was dissolved in water via a 50 ml volumetric flask. Co 3 O 4 nanorods (0.80 g) was dispersed in 50.0 g deionized water with strong agitation to make a homogeneous black suspension. The prepared Rh(NO 3 ) 3 aqueous solution was added by micropipette to the suspension of dispersed Co 3 O 4 nanorods. Vigorous stirring for 1 h is necessary to make sure a homogeneous distribution and preliminary natural adsorption of Rh 3+ on the surface of Co 3 O 4 nanorods. The pH was then gradually adjusted to 9.0 by ammonium hydroxide solution monitored with a pH meter. After that, the solution was stirred vigorously for another 12 h to reach an equilibrium for a thorough, homogeneous adsorption of Rh 3+ ions and followed by washing with deionized water and centrifuged. The catalyst precursor was dried in vacuum at 70 °C for at least 12 h. Then it was oxidized and reduced at an appropriate temperature so that the singly dispersed bimetallic site Rh 1 Co 3 can be prepared. Synthesis of Rh–Co bimetallic nanoparticles supported on CoO and Rh–Co alloy nanoparticles/SiO 2 (Rh: 5 wt%) was achieved by aqueous impregnation of Rh and Co precursors to SiO 2 NPs or Co 3 O 4 nanorods. Rh(NO 3 ) 3 ˙ x H 2 O (Sigma-Aldrich, ∼ 36% Rh basis) and Co(NO 3 ) 3 ˙6H 2 O (Sigma-Aldrich, ≥98%) were used as precursors of Rh and Co, respectively. The total weight per cent of Rh and Co is 5 wt% while keeping the atomic ratios of the loaded Rh and Co identical. Rh(NO 3 ) 3 ˙ x H 2 O and Co(NO 3 ) 2 ˙6H 2 O were dissolved in deionized water to make a clear solution. SiO 2 (0.5 g) or Co 3 O 4 nanorods (0.5 g) were immersed into the solution. The water was gradually evaporated at 60 °C with vigorous stirring and the catalyst was then dried in vacuum at 60 °C for 12 h, followed by calcination in 5% O 2 at 150 °C for 3 h. Before catalytic measurement, the catalyst was pretreated at 300 °C in 5% H 2 . Rh 1 O n /CoO was synthesized by introduction of Rh cations to well-prepared CoO by deposition–precipitation with a following annealing in N 2 and then a reduction at 200 °C in 5% H 2 for 1 h. In situ studies using ambient pressure X-ray photoelectron spectroscopy In situ studies of surface chemistry of these catalysts were performed on the ambient pressure XPS using monochromated Al Kα in the Tao group [11] , [29] , [30] . The binding energy of catalyst samples were calibrated to Au 4 f 7/2 at 84.0 eV and Ag 3 d 5/2 at 368.3 eV (ref. 11 ). In the AP-XPS studies, one or more reactant gases were introduced into a reactor. A sample is inserted and placed at the cross point of Rowland cycle of the monochromator and trajectory line of photoelectrons in lens of differentially pumped energy analyser. A distance between sample surface and the aperture of pre-lens of the differential pumping stage remains at ∼ 0.5 mm, which is shorter than the mean free paths of photoelectrons travelling in a gaseous environment of 5 Torr. Measurements of catalytic performance for reduction of NO with CO Reduction of NO with CO on catalysts is performed in a fixed-bed flow reactor. Gas computations and flow rates were marked in captions of figures. Details of catalytic measurement using our fixed-bed flow reactor can be found in our previous publications [9] , [10] . In situ studies using XANES and EXAFS In situ X-ray absorption spectroscopy (XANES) measurements were performed at the beamline X18B at the National Synchrotron Light Source, Brookhaven National Laboratory. The samples were made by pressing the powders into circular pellets using hydraulic press and transferred onto a sample holder of a Nashner–Adler in situ cell [31] . The data in the XANES region of the absorption coefficient were analysed by applying the same procedure for pre-edge line fitting, post-edge curve fitting and edge-step normalization to all the data. The XANES and extended X-ray absorption fine structure (EXAFS) data processing and analysis were performed using the IFEFFIT package [32] . The EXAFS data modelling and analysis were performed using standard procedures [32] , [33] , [34] , [35] , [36] . Computational methods The calculations were performed with the Vienna Ab-initio Simulation Package (VASP version 5.2). Both (011) and (001) surfaces of cobalt monoxide were represented by a periodic slab model constructed using bulk cell dimensions: a = b = c =4.2667 Å (ref. 37 ). Only calculation results of (011) surface were described in the main text. Since CoO is antiferromagnetic and has atomic moment on cobalt atoms, the primitive cubic unit cell of CoO was used to build the surface slab, which was previously proved to be the most energetically stable configuration for CoO [38] . The repeated slabs were separated from their neighbouring images by a 12 Å-width vacuum in the direction perpendicular to the surface. Considering the usually very large relaxations of the CoO surfaces, a slab containing five layers of 60 atoms was chosen. The three top-layer slabs of the surface were allowed to relax while the other layers beneath the surface were frozen during the geometry optimization ( Supplementary Fig. 10 ). The core and valence electrons were represented by the projector-augmented wave method and plane-wave basis functions with a kinetic energy cut-off of 400 eV. Inasmuch as Rh has non-negligible relativistic effects, the mass–velocity and Darwin relativistic effects were included through the projector-augmented wave potentials. The generalized gradient approximation with the Perdew–Burke–Ernzerhof exchange-correlation functional was used in the calculations. A Monkhorst–Pack grid of size of 2 × 2 × 1 was used to sample the surface Brillouin zone. Ground-state atomic geometries were obtained by minimizing the forces on the atoms to <0.02 eV Å −1 . Because of the strong d -electron correlation effects for Co, the calculations were carried out with the DFT+U method. The parameters were set at U =4 eV and J =1 eV according to previous reports [39] and our investigation ( Supplementary Tables 5, 6 ). The transition states were obtained by relaxing the force <0.02 eV Å −1 by using the dimer method [40] . How to cite this article: Zhang, S. et al. Catalysis on singly dispersed bimetallic sites. Nat. Commun. 6:7938 doi: 10.1038/ncomms8938 (2015).